Modern Antarctic acorn worms form tubes Acorn worms, or enteropneusts, are vermiform hemichordates that occupy an important position in deuterostome phylogeny. Allied to pterobranch hemichordates, small colonial tube dwellers, modern enteropneusts were thought to be tubeless. However, understanding of hemichordate diversity is poor, as evidenced by absence of reports from some oceanic regions and recent descriptions of large epibenthic deep-water enteropneusts, Torquaratoridae. Here we show, based on expeditions to Antarctica, that some acorn worms produce conspicuous tubes that persist for days. Interestingly, recent fossil descriptions show a Middle Cambrian acorn worm lived in tubes, leading to speculation that these fossils may have been pterobranch forbearers. Our discovery provides the alternative interpretation that these fossils are similar to modern-day torquaratorids and that some behaviours have been conserved for over 500 million years. Moreover, the frequency of Antarctic enteropneusts observed attests to our limited knowledge of Antarctic marine ecosystems, and strengthens hypotheses relating more northern deep-sea fauna to Antarctic shelf fauna. Hemichordates occur from intertidal to abyssal depths of the ocean and are important for understanding deuterostome phylogeny [1] , [2] , [3] . In particular, hemichordates with their sister group, echinoderms, form Ambulacraria [1] , and provide insights into the deuterostome ancestor. The two major body plans within hemichordates are the tube-dwelling Pterobranchia and the vermiform Enteropneusta or acorn worms. Acorn worms are notoriously difficult to collect intact as their long slender bodies are very soft and usually fragment on collection. Because of these sampling difficulties, until recently, enteropneusts were poorly known from the deep sea. Increased application of deep-sea imaging has helped alleviate this problem and resulted in description of a new family of deep-sea enteropneusts, Torquaratoridae [4] , [5] . Further, reports of enteropneusts from the Antarctic region have been limited to brief mentions in ecological studies [6] , [7] , [8] . Herein we report the discovery of large tube-dwelling acorn worms from the Antarctic. Deep-sea imaging techniques allowed documentation of several individuals of two different enteropneust morphotypes in mucous tubes. Phylogenetic analyses of ribosomal genes obtained from tissue fragments verified that these worms were allied to Torquaratoridae. Our results suggest that the recently described Middle Cambrian Spartobranchus tenuis [9] may be allied to modern enteropneusts. Enteropneust discovery During oceanographic cruises between 2008 and 2013, enteropneusts were imaged and partial animals collected by Blake trawl from Antarctic continental shelf regions at depths ranging from 531 to 1,111 m ( Fig. 1 ). Our imaging and collection efforts focused along the West Antarctic Peninsula shelf and adjacent fjords and on the Ross Sea shelf. At least two mobile, epibenthic morphotypes of acorn worms were observed forming meandering tracts on the ocean floor, and range in size up to 60 cm in length and 12 cm in width. Most individuals possessed a broad collar region and an overall morphology similar to that of torquaratorids. This designation was further confirmed by ribosomal RNA phylogenetic analysis of fragments from two individuals collected in the Ross Sea ( Fig. 2 ). One worm was sister to all other torquaratorids and neither were closely related to known species. 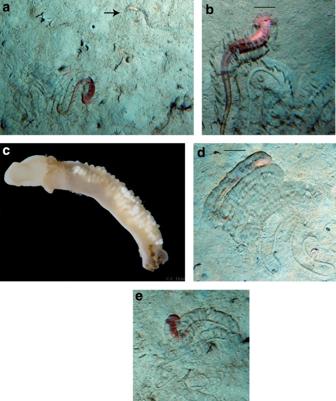Figure 1: Antarctic enteropneusts. (a) YoYo camera image of two morphotypes observed in the Ross Sea showing mucous-like tube. Pale morphotype denoted by arrow. (b). Large purple morphotype in secreted tube with proboscis expanded. (c) Pale morphotype worm similar to worm in upper right ofFig. 1a. and Antarctic sp. 1 (H89.3R) inFig. 2. Photo credit: Christoph Held. (d) Worm in tube made after zigzagging crawling pattern. (e) Worm showing ridges of sediment on tube. Scale bars, 10 cm (b,d). Figure 1: Antarctic enteropneusts. ( a ) YoYo camera image of two morphotypes observed in the Ross Sea showing mucous-like tube. Pale morphotype denoted by arrow. ( b ). Large purple morphotype in secreted tube with proboscis expanded. ( c ) Pale morphotype worm similar to worm in upper right of Fig. 1a . and Antarctic sp. 1 (H89.3R) in Fig. 2 . Photo credit: Christoph Held. ( d ) Worm in tube made after zigzagging crawling pattern. ( e ) Worm showing ridges of sediment on tube. Scale bars, 10 cm ( b , d ). 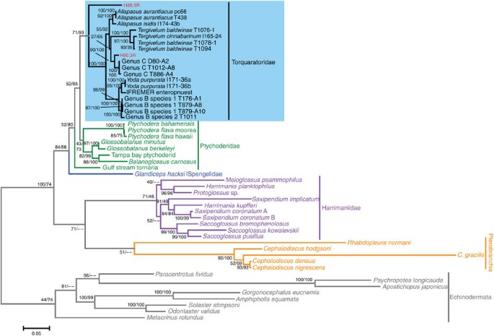Figure 2:18Shemichordate phylogeny. Maximum likelihood tree produced with the GTR+I+G model. Nodal values represent percentage support for a given node out of 5,000 bootstrap iterations. ‘Antarctic sp. 1 H89.3R’ is similar to the worm inFig. 1c. ‘Antarctic sp. 2 H90.3R’ was more pinkish in colour. Both worms were from the Ross Sea (76°20.473′S, 170°51.029’W) collect at 531 m depth. Full size image Figure 2: 18S hemichordate phylogeny. Maximum likelihood tree produced with the GTR+I+G model. Nodal values represent percentage support for a given node out of 5,000 bootstrap iterations. ‘Antarctic sp. 1 H89.3R’ is similar to the worm in Fig. 1c . ‘Antarctic sp. 2 H90.3R’ was more pinkish in colour. Both worms were from the Ross Sea (76°20.473′S, 170°51.029’W) collect at 531 m depth. Full size image Tube morphology Incredibly, most worms were imaged in translucent tubes secreted by the worms. Tubes generally appear to be attached to the worm along the posterior region of the collar ( Fig. 1a,b,e ) consistent with tube secretion occurring from specialized organs or tissue at the base of the collar. As we were limited to dredge sampling, none of the collected animals retained their tube, and the soft-bodied worms were in poor condition. Thus, we were unable to confirm the composition of the tubes or thoroughly address morphology. Fortunately, time-lapse photographs ( Fig. 3 and Supplementary Movie 1 ) taken in show one worm next to a recently vacated tube [8] . Aspects of the tube are still visible 60 h later. 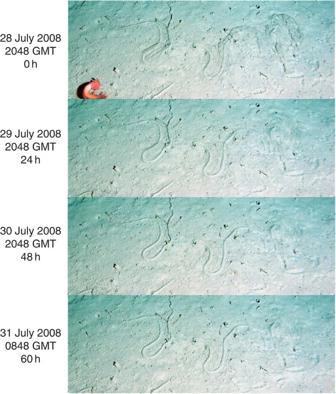Figure 3: Persistence of enteropneust tube. Using a time-lapse camera, images of an enteropneust and its tube were obtained at 12-h intervals starting 2048 GMT 28 July 2008 until 2048 GMT 2 August 2008. Figure panels show the tube over a 60-h period. The camera was located on the west Antarctic Peninsula shelf floor at Station B (64°46.420′S, 65°23.669′W) at a depth of 599 m. SeeSupplementary Movie 1 Figure 3: Persistence of enteropneust tube. Using a time-lapse camera, images of an enteropneust and its tube were obtained at 12-h intervals starting 2048 GMT 28 July 2008 until 2048 GMT 2 August 2008. Figure panels show the tube over a 60-h period. The camera was located on the west Antarctic Peninsula shelf floor at Station B (64°46.420′S, 65°23.669′W) at a depth of 599 m. See Supplementary Movie 1 Full size image Until the observations here, extant enteropneusts were not known to produce or live in large secreted mucous tubes. By contrast, pterobranchs (including graptolites) can make extensive and elaborate secreted tube systems. Thus, discovery of large tubicolous enteropneusts from the Antarctic is significant for multiple reasons. Foremost, our discovery provides context for the recently re-described Middle Cambrian fossils [9] , S. tenuis from the Burgess Shale Formation. These acorn worm fossils look remarkably like present-day enteropneusts, except many are observed to be within a ‘fiberous’tube. The persistence of tubes in Antarctic worms suggests that the tubes contain proteinaceous components functioning as binding agents. Some tubes were lightly covered with sediment giving them a ‘ribbed’ appearance, similar to those reported for S. tenuis (compare Fig. 1e with ref. 9 Fig. 2b,c). Observations in ref. 9 include helical, branched and circular tubes, and they further suggest that the worms could abandon their tubes [9] . Our observations of Antarctic tubicolous worms and faecal casings imply that the worms often turn and zigzag during movement or may even double back on themselves as reported elsewhere [10] , [11] . If buried quickly in a single obtrusion event, as suspected for each of the mudstone beds of the Greater Phyllopod Bed (that is, Walcott’s quarry) [12] , such tubes could appear helical or even circular as reported for S. tenuis . (note: worms occupying a circular tube, as hypothesized in ref. 9 , would present problems for feeding, defecation and possibly respiration). The fossil tubes were interpreted as ‘fiberous’ based on apparent tearing of the tubes, but a similar phenomenon occurs with the present-day tubes ( Fig. 3 and Supplementary Movie 1 ). Given the similarity in tube design between S. tenuis and the Antarctic torquaratorids, similar behavioural repertoires (for example, tube building, vacating tubes and meandering epibenthic movements) appear to have been conserved ~500 million years. Given the presence of tubes in modern toraquaratorid worms, we hypothesize that S. tenuis is probably allied to torquaratorids rather than to pterobranch-harrimaniid ancestors [9] . Fossil evidence [13] , [14] , [15] reveals that graptolites, and even rhabopleurids and cephalodiscids (modern pterobranch lineages), were present in the Middle Cambrian, making S. tenuis contemporary with established pterobranch (including graptolite) lineages. As the split between enteropneust and pterobranch lineages would have been before the Middle Cambrian, the tube of S. tenuis was not a precursor to the pterobranch coenecium. Lack of synapticulae and hepatic sacs were also argued to ally S. tenuis with harrimaniid enteropneusts. However, torquaratorid enteropneusts, like harrimaniids, lack synapticles [4] , and assessing the presence of hepatic sacs often requires microscopy in modern species, much less in fossilized ones. Given the position of torquaratorids and pterobranchs in hemichordate phylogeny, the last common hemichordate ancestor may have been able to build tubes, raising the question whether this ability was present in the last common deuterostome ancestor. This discovery also has important implication for Antarctic science. The torquaratorids reported here are the shallowest on record, discovered on the Antarctic shelf at 531 m, whereas previous reports in northern latitudes are from 1,600 to 4,000 m. Our observations of Protelpida and Peniagone (deep-sea holothuroids) along with torquarartorids on the Antarctic shelf bolster hypotheses of a close connection between Antarctic shelf fauna and deep-sea fauna [16] , [17] . Before this submission, the class Enteropneusta was essentially unknown from most of the Antarctic region, yet on our expeditions, they were repeatedly observed in camera transects on the continental shelf in east and west Antarctica [8] . These results underscore how poorly the biodiversity of Antarctic shelf fauna is known [18] and that more effort is needed to understand this rapidly changing region. Imaging Scientific research expeditions were aboard the RVIB Nathaniel B. Palmer in 2008 to the Antarctic Peninsula and 2013 to the Ross Sea. Sea floor imaging used a vertically oriented YoYo camera system comprised an ocean imaging systems (OIS) DSC 10,000 digital still camera with an OIS 3831 strobe that was triggered by a bottom contact switch 2.5 m above the bottom to render an ~3 m 2 image of the sea floor [8] . Parallel laser beams set at 10 cm apart provided the scale. The camera system was repeatedly raised and lowered, to trigger the bottom contact, as the ship held course at approximately 1 knot. The time-lapse system employed the same OIS camera and strobe system described above deployed on the seafloor on an aluminium tripod with the camera elevation of 163 cm and a camera angle from horizontal (inclination) of 45°. The interval between photos in the time-lapse mode was 12 h. The time-lapse camera was located on the west Antarctic Peninsula shelf floor at Station B (64°46.420′S, 65°23.669′ W) at a depth of 599 m. Images of the enteropneust and its tube were obtained from 28 July to 2 August 2008. Molecular analyses Benthic samples were obtained from the Ross Sea by a Blake trawl with a 2-m opening. Sampled were sorted and preserved on deck. Sequencing and phylogenetic protocols of 18S and 16S ribosomal DNA used the standard procedures [3] . PCR amplification used primers 16Sar 5′-CGCCTGTTTATCAAAAACAT-3′ and 16Sbr 5′-CCGGTCTGAACTCAGATCACGT-3′ for 16S ribosomal DNA and 18e 5′-CTGGTTGATCCTGCCAGT-3′ and 18 P 5′-TAATGATCCTTCCGCAGGTTCACCT-3′. Supplementary Table S1 provides GenBank Accession numbers for taxa used herein, and the matrix is in Supplementary Data 1 . Maximum likelihood and Bayesian analyses (both used the best fitting model GTR+I+G) were conducted with RaxML version 7.3.9 (ref. 19 ) (5,000 bootstrap replicates) and MrBayes version 3.2.0 (ref. 20 ) (four independent runs for 5,000,000 generations sampled every 100 generations), respectively. Accession codes: Novel capillary sequence data were deposited in GenBank nucleotide database under Accession numbers KF683552 , KF683558 , KF683564 and KF683573 . How to cite this article: Halanych, K. M. et al . Modern Antarctic acorn worms form tubes. Nat. Commun. 4:2738 doi: 10.1038/ncomms3738 (2013).